Interaction between prion protein and toxic amyloid β assemblies can be therapeutically targeted at multiple sites A role for PrP in the toxic effect of oligomeric forms of Aβ, implicated in Alzheimer's disease (AD), has been suggested but remains controversial. Here we show that PrP is required for the plasticity-impairing effects of ex vivo material from human AD brain and that standardized Aβ-derived diffusible ligand (ADDL) preparations disrupt hippocampal synaptic plasticity in a PrP-dependent manner. We screened a panel of anti-PrP antibodies for their ability to disrupt the ADDL–PrP interaction. Antibodies directed to the principal PrP/Aβ-binding site and to PrP helix-1, were able to block Aβ binding to PrP suggesting that the toxic Aβ species are of relatively high molecular mass and/or may bind multiple PrP molecules. Two representative and extensively characterized monoclonal antibodies directed to these regions, ICSM-35 and ICSM-18, were shown to block the Aβ-mediated disruption of synaptic plasticity validating these antibodies as candidate therapeutics for AD either individually or in combination. Soluble non-fibrillar forms of amyloid β-protein (Aβ) have been implicated in, and shown to correlate with, disease progression in animal models of Alzheimer's disease (AD) and patients with AD [1] . Low nanomolar concentrations of synthetic Aβ are known to disrupt synaptic plasticity in vivo and in vitro , but the conformation and size of the Aβ species responsible remain unclear [2] , [3] , [4] , [5] . It has recently been reported that the prion protein (PrP C ) can function as a cellular receptor for a preparation of synthetic Aβ referred to as Aβ-derived diffusible ligands (ADDLs) and that PrP C is required for the disruption of synaptic plasticity mediated by ADDLs [6] . Nanomolar affinity of binding has been reported [7] , [8] , [9] and a single anti-PrP monoclonal antibody with an epitope around residues 95–105 blocked ADDL binding and toxicity [6] . In further studies, constitutive knockout of PrP C expression reversed several pathological phenotypes in a mouse model of AD [10] as did peripheral treatment of the same mouse model with an anti-PrP antibody [11] . If confirmed, such a finding is of considerable importance given the extensive investigation of targeting PrP C for prion disease therapeutics [12] . In particular, the abolition of neuronal PrP expression in the adult murine nervous system is without serious consequence [13] , [14] and both small molecule [12] and monoclonal antibody therapeutics [15] have been extensively studied. Indeed therapeutic molecular interactions with PrP C have been characterized and fully humanized anti-PrP monoclonal antibodies have been produced for clinical studies in human prion disease [16] , [17] . However, a number of groups have since reported deleterious effects of Aβ that do not require PrP expression [7] , [8] , [18] . In this context, it is important to recognize that a range of different Aβ preparations have been used and that this may in part explain some of the conflicting reports. Moreover, discrepancies between animal, tissue, cellular and biochemical AD models with respect to a possible role for PrP C are to be anticipated. AD is a heterogeneous disease and perhaps better considered to be a clinicopathological syndrome with multiple genetic and environmental factors involved in its aetiology and progression. The many reported animal models of AD each recapitulate only part of this syndrome. Even if PrP C is indeed an important receptor for toxic Aβ species, it would not be reasonable to expect PrP C ablation to rescue all aspects of pathology in each model. Further, given that the concentration of the active species is not known and may differ between studies by different groups some effects may be due to higher Aβ concentrations, which could elicit nonspecific toxic effects. We first sought to repeat the studies of Laurén et al . [6] on synaptic plasticity, using congenic wild-type and PrP null lines, to confirm the PrP-dependence of the toxicity of our ADDLs and to characterize the putative PrP:Aβ interaction. Given the poor characterization and variable toxicity of different Aβ preparations, we were careful to use only formulations which caused impairment of long-term potentiation (LTP) and conformed to defined biophysical criteria consistent with previous descriptions of ADDLs [3] , [6] , [19] . However, as it is unclear whether Aβ species similar to those found in ADDL preparations are present in human brain, we considered it essential to also determine if PrP C was required for the synaptic plasticity-impairing effects of AD brain-derived Aβ. Thereafter, we proceeded to further studies aimed at characterization of the putative therapeutic target and approaches to block PrP:Aβ interaction and its effects on synaptic plasticity. We confirmed that well-characterized ADDL preparations inhibit LTP in a PrP-dependent manner and that the block of LTP mediated by the most disease-relevant form of Aβ, Aβ extracted from AD brain, requires expression of PrP. We also report the development of a high-throughput screen, which allowed us to identify antibodies that recognize certain epitopes contained both within and outside the previously characterized Aβ:PrP-binding site. Notably, antibodies to helix-1 of PrP, prevented ADDL binding to PrP and the block of LTP mediated by both ADDLs and AD brain-derived Aβ. Characterization of reproducible preparations of ADDLs We used a standardized procedure to generate ADDL preparations from Aβ 1−42 or bADDL preparations from biotinylated Aβ 1−42 (bAβ 1−42 ) and then assessed the consistency of the species produced using a battery of biophysical tests. Both unmodified and biotinylated Aβ were used to confirm that biotinylation did not fundamentally alter the properties of the oligomers. Size-exclusion chromatography (SEC) using three different running buffers showed that both ADDLs and bADDLs had highly similar profiles producing two prominent peaks ( Fig. 1a ; Supplementary Fig. S1 ). The first peak eluted in the void volume and the second eluted in a volume consistent for Aβ monomer [20] . Moreover, both peaks had trailing and leading shoulders suggesting the presence of low abundance oligomers intermediate in size between Aβ monomer and the void material. Given the limited size resolution of SEC, and the possibility of forming artefacts owing to non-ideal interactions with the column, we also analysed our bADDL preparations using a solution-based technique, analytical ultracentrifugation (AUC) ( Fig. 1b ). Sedimentation of bADDLs occurred in two distinct phases containing ∼ 60 and 40% of the material, respectively. The initial sedimentation contained a mixture of species with calculated masses ranging from 90 to 400,000 and accounted for around 60% of the peptide. The slowly sedimenting portion contained a single species with calculated molecular weight of 5–6,000 close to the value expected for monomeric, biotinylated Aβ peptide. In agreement with the SEC results, the AUC data confirm that bADDL preparations are heterogeneous and include Aβ monomer, small amounts of low n -oligomers and species with calculated masses >90,000. It is noteworthy that in all samples tested bADDL preparations contained slightly greater amounts of high-molecular-weight species than did ADDLs ( Fig. 1a ; Supplementary Fig. S1 ). Consistent with other biophysical assessments, negative-stain electron microscopy (EM) confirmed that ADDL and bADDL preparations contained a mixture of different sized species, ranging from globular structures of 8–12 nm diameter and flexible rods of 15–60 nm in length and 5–10 nm diameter ( Fig. 1c,d ; Supplementary Fig. S2 ). These structures are reminiscent of those detected by Laurén et al . [6] , but are in contrast to the entirely globular structures observed by Chen et al . [9] and Balducci et al . when prepared using simple phosphate buffer [7] . The species detected by SEC, AUC and EM were SDS-labile and migrated on SDS–PAGE predominantly as monomer ( Fig. 1e,f ), however, a small amount of higher molecular weight Aβ species were detected if samples were not boiled before SDS–PAGE and proteins visualized by western blotting. As a major factor which we have found to influence production of ADDL preparations of consistent composition is the effective solubilization of hexafluoro-2-propanol (HFIP)-treated Aβ, we used SDS–PAGE and silver staining as a simple means to measure the total amount of Aβ present in all our ADDL preparations. These experiments revealed that the actual concentration of total Aβ in our ADDL preparations varied between 70 to 90 μM (based on the molecular weight of Aβ monomer), less than the 100 μM concentration based on the starting amount of Aβ used. 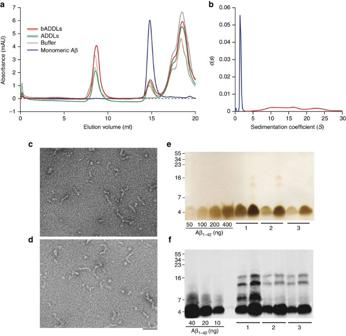Figure 1: Biophysical characterization of Aβ species present in the bADDL preparation. (a) Size-exclusion chromatography of two different batches of freshly prepared ADDLs and bADDLs eluted in PBS showing the ratio of oligomeric (left) to monomeric (middle) Aβ, as well as a buffer peak (right). (b) Velocity analytical ultra centrifugation of freshly prepared bADDLs in Ham's F12 medium as detected by absorbance at 280 nm and represented by continuous distributionc(s), the sedimentation coefficient distribution. The monomer (calculated molecular mass 5,000–6,000) and the oligomer components (calculated molecular mass 90,000–400,000) have been coloured blue and red, respectively. (c,d) Negatively stained transmission electron micrograph of (c) bADDLs and (d) ADDLs showing a mixture of globular and rod-like structures <100 nm in length. Scale bar, 50 nm. (e,f) SDS–PAGE of ADDL preparations analyzed by silver staining (e) to estimate the amount of soluble Aβ present in three different ADDL preparations (labelled 1, 2 and 3) and western blot analysis (f) using the N-terminal anti-Aβ antibody, 6E10, to identify low abundance SDS-stable Aβ species. Two different concentrations of each test sample (10 μM and 20 μM, for Silver stain and 1 μM and 2 μM for western blot) were examined. Figure 1: Biophysical characterization of Aβ species present in the bADDL preparation. ( a ) Size-exclusion chromatography of two different batches of freshly prepared ADDLs and bADDLs eluted in PBS showing the ratio of oligomeric (left) to monomeric (middle) Aβ, as well as a buffer peak (right). ( b ) Velocity analytical ultra centrifugation of freshly prepared bADDLs in Ham's F12 medium as detected by absorbance at 280 nm and represented by continuous distribution c ( s ), the sedimentation coefficient distribution. The monomer (calculated molecular mass 5,000–6,000) and the oligomer components (calculated molecular mass 90,000–400,000) have been coloured blue and red, respectively. ( c , d ) Negatively stained transmission electron micrograph of ( c ) bADDLs and ( d ) ADDLs showing a mixture of globular and rod-like structures <100 nm in length. Scale bar, 50 nm. ( e , f ) SDS–PAGE of ADDL preparations analyzed by silver staining ( e ) to estimate the amount of soluble Aβ present in three different ADDL preparations (labelled 1, 2 and 3) and western blot analysis ( f ) using the N-terminal anti-Aβ antibody, 6E10, to identify low abundance SDS-stable Aβ species. Two different concentrations of each test sample (10 μM and 20 μM, for Silver stain and 1 μM and 2 μM for western blot) were examined. Full size image AD brain-derived Aβ inhibits LTP in a PrP-dependent manner Having established procedures to produce and characterize our bADDL and ADDL preparations, we sought to assess their effect on synaptic plasticity and to determine whether this effect required expression of PrP. As expected, both our bADDL and ADDL preparations significantly inhibited LTP in hippocampal slices from wild-type FVB/N and C57Bl/6J mice ( P <0.01, one-way analysis of variance (ANOVA), Fig. 2a ; Supplementary Fig. S3 ). Using an FVB/N congenic PrP null mouse line we next investigated whether this Aβ-mediated inhibition of LTP required the expression of PrP. As in a previous study using another PrP null mouse model [6] , bADDLs that blocked LTP in wild-type mice failed to impair LTP in the hippocampi of our PrP null mice ( Fig. 2b ). Although these results suggest a potential role for PrP in bADDL-mediated depression of hippocampal LTP, it is not clear if such preparations include Aβ species that occur in AD brain. Therefore, we sought to determine whether water-soluble extracts of AD brain that contain SDS-stable Aβ dimers also required the expression of PrP for their plasticity-impairing effects. For these experiments, we used a brain extract from a non-demented control subject that lacked detectable Aβ and a Tris-buffered saline (TBS) extract from an AD brain that contained significant amounts of Aβ monomer and SDS-stable dimer ( Fig. 2c ). As in earlier experiments [21] , the Aβ-containing extracts potently inhibited LTP in slices from FVB/N mice ( Fig. 2d , P <0.01, one-way ANOVA), whereas TBS extracts that lacked Aβ had no effect ( Fig. 2d ). Importantly, as was the case with bADDLs ( Fig. 2b ), the block of LTP mediated by brain-derived Aβ required the expression of PrP C , with the AD-TBS extract unable to alter LTP in hippocampal slices from PrP null mice ( Fig. 2d ). As expected, application of TBS extract from a control brain, that lacked detectable amounts of Aβ, had no effect on LTP in slices from either PrP expressing or PrP null FVB/N mice ( Fig. 2d and 168±10% versus 164±10%, respectively). These findings provide important evidence that PrP is required for the plasticity-impairing effects of pathogenically relevant brain-derived Aβ species and suggest that PrP may be required for the changes in synaptic function that characterize the earliest stages of AD [22] . As yet, it is unclear as to how the active Aβ species in human brain relate to the active species present in an Aβ preparation such as ADDLs. It is worth pointing out that both sources are heterogenous, ADDLs contain a mixture of different sized Aβ species ranging from monomer to ∼ 2 MDa [19] and the water-soluble extract of AD brain contains Aβ ranging from monomer to ≥70 kDa [21] . In the case of water-soluble brain extracts, fractions rich in SDS-stable dimers have been shown to mediate synaptotoxicity, however, whether this activity is mediated by discrete Aβ dimers, or assemblies built from SDS-stable dimers is not clear [21] , [23] . Indeed, we have recently shown that synthetic Aβ dimers alone are not synaptotoxic, but must assemble into larger pre-fibrillar Aβ structures to perturb synaptic plasticity [23] . Thus, although we cannot yet provide a direct comparison of the biophysical properties of brain-derived Aβ and the polydisperse collection of assemblies that constitute ADDLs, it is remarkable that both ADDLs and human brain-derived Aβ require the expression of PrP to exert their toxic effects. 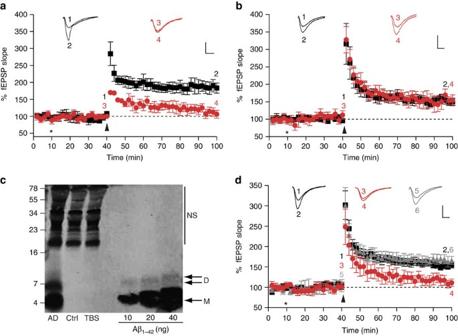Figure 2: PrPCis required for the inhibition of LTP by bADDLs and Aβ-containing extracts of human brain. fEPSPs were recorded from the CA1 region of the hippocampus in all cases. Insets show example fEPSP traces before and 1 h post theta-burst (TB) stimulation (stimulus artefact was removed for clarity).Pvalues were calculated using one-way ANOVA and the Tukey–Kramerpost hoctest. (a) Extracellular recordings from FVB/N mice show stable LTP measured up to 1 h post-TB (black squares, 184±15%,n=7). Pretreatment of the slices with bADDLS for 30 min before TB caused a significant inhibition of LTP (red circles, 109±10%,P<0.01,n=6). (b) LTP was reliably induced in slices from PrP null mice treated with vehicle control (black squares, 151±8%,n=6). Significantly, perfusion of slices from PrP null mice with the same bADDL preparation used ina, did not impair LTP (red circles, 149±11%,n=5,P>0.05). (c) Immunoprecipitation/western blot analysis of brain extracts revealed the presence of abundant Aβ monomer (M) and SDS-stable dimer (D) in a sample taken from an AD brain and the complete absence of Aβ in an extract from a non-demented control subject (Ctrl). Estimates of Aβ concentration indicate the presence of 14 and 3.2 ng ml−1of monomer and SDS-stable dimer, respectively. Nonspecific (NS) immunoreactive bands were detected when Tris-buffered saline (TBS) alone was immunoprecipitated. Molecular weight markers are on the left. (d) Perfusion of slices from wild-type FVB mice with AD brain for 30 min before TB significantly impaired LTP (red circles, 116±9%,n=6) compared with slices perfused with control brain extract (black squares, 153±8%,n=6,P<0.05). In contrast, treatment of slices from PrP−/−mice with AD brain extracts failed to alter LTP (grey triangles, 164±10%,n=6,P>0.05). *Refers to when perfusion of bADDLs/AD brain extract was started and arrow denotes application of TB. The numbers on the example EPSPs (insets) represent the time points of the average fEPSP slope values indicated with the same numbers. All values are mean±s.e.m. Scale bar on insets denotes 1 mv, 5 ms. Figure 2: PrP C is required for the inhibition of LTP by bADDLs and Aβ-containing extracts of human brain. fEPSPs were recorded from the CA1 region of the hippocampus in all cases. Insets show example fEPSP traces before and 1 h post theta-burst (TB) stimulation (stimulus artefact was removed for clarity). P values were calculated using one-way ANOVA and the Tukey–Kramer post hoc test. ( a ) Extracellular recordings from FVB/N mice show stable LTP measured up to 1 h post-TB (black squares, 184±15%, n =7). Pretreatment of the slices with bADDLS for 30 min before TB caused a significant inhibition of LTP (red circles, 109±10%, P <0.01, n =6). ( b ) LTP was reliably induced in slices from PrP null mice treated with vehicle control (black squares, 151±8%, n =6). Significantly, perfusion of slices from PrP null mice with the same bADDL preparation used in a , did not impair LTP (red circles, 149±11%, n =5, P >0.05). ( c ) Immunoprecipitation/western blot analysis of brain extracts revealed the presence of abundant Aβ monomer (M) and SDS-stable dimer (D) in a sample taken from an AD brain and the complete absence of Aβ in an extract from a non-demented control subject (Ctrl). Estimates of Aβ concentration indicate the presence of 14 and 3.2 ng ml −1 of monomer and SDS-stable dimer, respectively. Nonspecific (NS) immunoreactive bands were detected when Tris-buffered saline (TBS) alone was immunoprecipitated. Molecular weight markers are on the left. ( d ) Perfusion of slices from wild-type FVB mice with AD brain for 30 min before TB significantly impaired LTP (red circles, 116±9%, n =6) compared with slices perfused with control brain extract (black squares, 153±8%, n =6, P <0.05). In contrast, treatment of slices from PrP −/− mice with AD brain extracts failed to alter LTP (grey triangles, 164±10%, n =6, P >0.05). *Refers to when perfusion of bADDLs/AD brain extract was started and arrow denotes application of TB. The numbers on the example EPSPs (insets) represent the time points of the average fEPSP slope values indicated with the same numbers. All values are mean±s.e.m. Scale bar on insets denotes 1 mv, 5 ms. Full size image PrP/ADDL interaction can be targeted at multiple sites Having established the requirement for PrP for the plasticity-impairing activity of both AD brain-derived Aβ and ADDLs, we then set out to investigate whether active preparations of Aβ bound to PrP. Previous characterization of the PrP:Aβ interaction has been carried out using preparations of synthetic Aβ that acted in a PrP-independent manner [7] , had not been shown to be toxic [8] , [9] or were studied at micromolar concentrations [7] , [9] . We probed the interaction using a high-throughput plate-based DELFIA (dissociation-enhanced lanthanide fluorescent immunoassay). A binding response between huPrP 23−231 and either bADDLs or ADDLs was detected at low nanomolar concentrations with apparent dissociation constants for total Aβ of 82±7 and 100±30 nM, respectively ( Fig. 3a ), with no indication of a tight-binding component (Methods). Given that the total concentration of Aβ present in our stock solution was on average 20% less than the 100 μM value derived from the weight of starting peptide powder, that a significant portion of the peptide remained as monomer ( Fig. 1a,b ), and that the molar concentration of Aβ oligomers must (because of their higher molecular weight) be lower than the concentration based on monomer content, it is evident that one or more of the species present in ADDL preparations binds PrP very tightly, probably in the picomolar range. In contrast, Aβ monomer exhibited no binding to PrP at concentration ≤3×10 −7 M ( Supplementary Fig. S4 ). Nonspecific oligomer binding to a background BSA surface was observed for both ADDLs and bADDLs when the concentration was raised from high nanomolar to low micromolar, highlighting the importance of probing this interaction in the nanomolar range using well-defined Aβ preparations. Moreover, the modest binding observed when micromolar concentrations of monomer were used likely resulted because spontaneous aggregation of Aβ occurs in this concentration range [23] and, once formed, such aggregates could bind to PrP. Consequently, all subsequent experiments were carried out using bADDLs at a concentration of 100 nM (monomer equivalent Aβ) where the most specific interaction could be measured. Given that both PrP [24] and Aβ [25] are known to contain high-affinity for copper-binding sites in relevant positions, the possibility that their interaction may be mediated by copper chelation was investigated. Addition of up to 10 mM EDTA did not change the level of bADDL binding ( Supplementary Fig. S5 ). At these concentrations, EDTA should be capable of displacing copper from both PrP and Aβ [26] thus excluding simple, nonspecific copper chelation as the mechanism for the PrP:Aβ interaction. 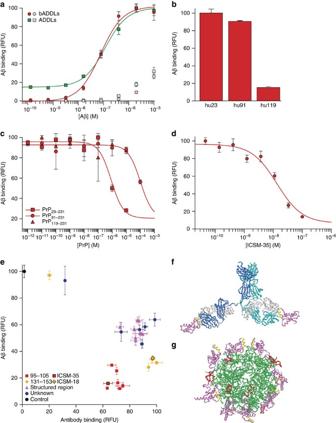Figure 3: bADDLs avidly bind PrP in a manner that can be blocked by certain anti-PrP antibodies. (a) Dose response curves of ADDLs (green) and bADDLs (red) to plate-bound full-length PrP or background wells coated with BSA (light green and red for ADDLs and bADDLs, respectively). (b) Binding of 100 nM bADDLs to huPrP23−231, huPrP91−231and huPrP119−231. (c) Competition of binding of bADDLs to surface-bound huPrP23−231by different constructs of PrP. (d) Inhibition of bADDL binding to huPrP23−231by ICSM-35 after pre-incubation of surface-bound huPrP23−231with ICSM-35. (e) Screen of the ICSM panel of antibodies using a high throughput DELFIA to detect bADDL or antibody binding. Antibodies are classed in different binding regions 95–105 (red), 131–153 (yellow), structured region (magenta) or undefined epitopes (blue). ICSM-18 and ICSM-35 are highlighted. Surface-bound huPrP23−231was pre-incubated for 1 h with 100 nM antibodies and then incubated for 1 h with or without 100 nM bADDLs before detection with either Eu-N1 streptavidin or Eu-N1 anti-mouse antibody. (f,g) Model of the PrP/ICSM-18 complex (f) based on the published crystal structure and with the antibody extension built in with PrP and the ICSM-18 epitope (yellow) highlighted; (g) Modelled structure of the PrP/Aβ interaction with Aβ spheroids (green), PrP (magenta), the ICSM-18 epitope (yellow) and the unstructured ICSM-35 epitope (red) built in, highlighting the large distance between Aβ-binding site and the ICSM-18 epitope. All graphs show mean±s.d. and are an average of at least three data points. Figure 3: bADDLs avidly bind PrP in a manner that can be blocked by certain anti-PrP antibodies. ( a ) Dose response curves of ADDLs (green) and bADDLs (red) to plate-bound full-length PrP or background wells coated with BSA (light green and red for ADDLs and bADDLs, respectively). ( b ) Binding of 100 nM bADDLs to huPrP 23−231 , huPrP 91−231 and huPrP 119−231 . ( c ) Competition of binding of bADDLs to surface-bound huPrP 23−231 by different constructs of PrP. ( d ) Inhibition of bADDL binding to huPrP 23−231 by ICSM-35 after pre-incubation of surface-bound huPrP 23−231 with ICSM-35. ( e ) Screen of the ICSM panel of antibodies using a high throughput DELFIA to detect bADDL or antibody binding. Antibodies are classed in different binding regions 95–105 (red), 131–153 (yellow), structured region (magenta) or undefined epitopes (blue). ICSM-18 and ICSM-35 are highlighted. Surface-bound huPrP 23−231 was pre-incubated for 1 h with 100 nM antibodies and then incubated for 1 h with or without 100 nM bADDLs before detection with either Eu-N1 streptavidin or Eu-N1 anti-mouse antibody. ( f , g ) Model of the PrP/ICSM-18 complex ( f ) based on the published crystal structure and with the antibody extension built in with PrP and the ICSM-18 epitope (yellow) highlighted; ( g ) Modelled structure of the PrP/Aβ interaction with Aβ spheroids (green), PrP (magenta), the ICSM-18 epitope (yellow) and the unstructured ICSM-35 epitope (red) built in, highlighting the large distance between Aβ-binding site and the ICSM-18 epitope. All graphs show mean±s.d. and are an average of at least three data points. Full size image The binding to different length constructs of PrP showed that huPrP 91−231 bound similar quantities of bADDLs, as did the full-length construct, suggesting the crucial high-affinity-binding site was not in the region 23–91 ( Fig. 3b ). In contrast, huPrP 119−231 displayed almost no binding, confirming the role of the 91–119 region in the high-affinity PrP:Aβ interaction. A competition assay, whereby increasing concentrations of the different PrP constructs were co-incubated with bADDLs to prevent binding to surface-bound huPrP 23−231 , confirmed that the interaction could occur in solution and revealed that while the region 23–90 did not appear to contain a separate high-affinity-binding site, it was indeed involved in modulating the high-affinity interaction ( Fig. 3c ). We then tested the ability of the antibody ICSM-35, which binds to an epitope contained in residues 95–105 of PrP [27] , the putative site of ADDL binding [6] for ability to block the PrP:Aβ interaction. This antibody blocked binding of bADDLs to PrP in a classical dose-dependent manner with an IC 50 =10.4±1.7 nM ( Fig. 3d ). A screen of 28 PrP-binding antibodies pre-incubated with PrP before the addition of bADDLs showed that all antibodies that bound fully to PrP were capable of blocking bADDL binding, at least in vitro , although their efficacy varied ( Fig. 3e ). The differences in efficacy were clearly epitope dependent, with those interacting directly with the putative ADDL-binding site most effective, followed by those that bind to helix-1 of PrP, whereas those binding to other structured regions of the protein were the least effective. There was no epitope-dependent correlation between the level of antibody binding and the level of inhibition, although, as expected, individual antibodies that failed to remain bound to PrP did not inhibit bADDL binding. Furthermore, the two best characterized antibodies that bind to helix-1 and the 95–105 epitope (ICSM-18 and ICSM-35, respectively), both bind to full-length human prion protein with affinities of ∼ 10 nM, block ADDLs with inhibition constants of ∼ 20 nM, yet still differ in the magnitude of their inhibition ( Supplementary Fig. S4 ). ICSM-18 and ICSM-35 were chosen for further characterization as representative members of the groups that bind to helix-1 and the 95–105 epitope, respectively, because of their proven efficacy as anti-prion therapeutics and they do not cause acute toxicity [15] . Moreover, the structure of the PrP:ICSM-18 complex has been solved at atomic resolution [16] . The ability of ICSM-18 to block the interaction, despite binding to an epitope far-removed from the 95–105 segment, is surprising ( Fig. 3f,g ). It is unlikely that the on-rate of PrP with the Aβ is reduced significantly by linking with the antibody, as the enlarged structure will diffuse only slightly more slowly. The dissociation rate of PrP from the Aβ structure is not likely to increase by linking interactions with the antibody owing to bulk-solvent effects. The antibody is also unlikely to cause disruption of the water structure or dielectric properties around the PrP:Aβ interface; hence, hydrophobic or electrostatic interactions will be largely unaffected. However, if PrP:PrP contact is needed to stabilize the PrP layer adhered to the Aβ aggregates, then interaction with the antibody would certainly prevent this and weaken the system. Multiple PrP-binding sites would suggest the bound Aβ assemblies contains a repeat structure. It may be that such antibodies prevent the binding of larger Aβ assemblies but not smaller species. Likewise, reorganization of the protein on the membrane surface could bring these epitopes into close proximity allowing ICSM-18 to sterically block the interaction, although this is unlikely to be the cause of the effect in a plate-based biochemical assay and would not explain the stronger inhibition of helix-1-directed antibodies compared with those that bind to structured areas closer to the Aβ oligomer-binding site. Either option opens up the possibility of using multiple antibodies to therapeutically block this interaction. Moreover, these results validate the use of this novel high throughput system as a useful first round screen to identify candidate therapeutics capable of inhibiting or modulating ADDL binding to PrP. Antibodies block the Aβ-mediated disruption of LTP in vivo To further assess the potential of two lead monoclonal antibodies identified in our screen, and that belong to the two groups of antibodies that most effectively blocked ADDL binding to PrP in vitro ( Fig. 3e ), we examined whether these antibodies could also block Aβ-mediated impairment of synaptic plasticity. To ensure the effect was not just present in FVB/N mice, this part of the study was carried out using hippocampal slices from C57Bl/6J mice. Perfusion of slices from C57Bl/6J mice with ADDLs 30 min before LTP induction significantly depressed LTP compared with slices treated with buffer control alone ( Fig. 4a , P <0.01, one-way ANOVA), whereas previous application of low concentrations of the anti-PrP antibody, ICSM-35 (2 μg ml −1 , 13 nM) abolished the ADDL-mediated impairment of LTP ( Fig. 4a , P <0.01, one-way ANOVA). Similarly, when slices were incubated with ICSM-18 20 min before ADDLs this antibody also protected against the ADDL-mediated block of LTP ( Fig. 4b , P <0.01, one-way ANOVA). Importantly, both ICSM-18 and ICSM-35 had no significant effect on LTP when administered alone ( Supplementary Fig. S6a,b ). ICSM-35 is directed against amino acids 93–102 of PrP C , which includes the Aβ:PrP-binding domain identified in this and previous studies [6] , whereas ICSM-18 selectively binds to helix-1 of PrP [16] . Thus, unlike ICSM-35, which should directly target the ADDL-binding site, ICSM-18 may act by hindering formation of the PrP:Aβ interaction. 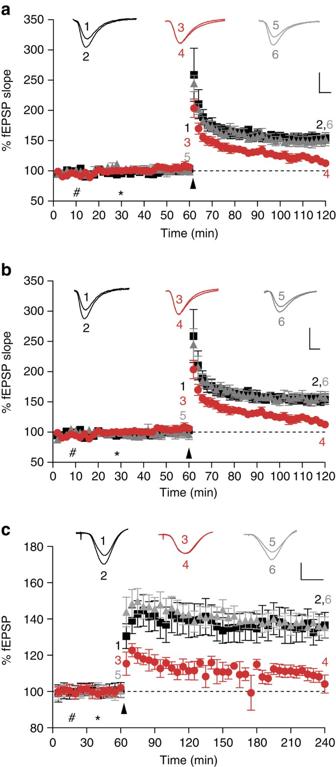Figure 4: Inhibition of LTP by ADDLs or Aβ-containing AD brain extract is ameliorated by the anti-PrPCantibodies ICSM-35 and ICSM-18. (a) Conditioning stimulation in hippocampal slices from C57Bl/6J mice treated with vehicle solution induced a robust LTP (black squares, 152±7%,n=6), whereas pretreatment (30 min) with ADDLs significantly depressed LTP (red circles, 115±5%,n=8, p<0.01). In contrast, perfusion of slices with the anti-PrP antibody, ICSM-35 (which recognizes an epitope within the residues 93–102; 2 μg ml−1), 20 min before application of ADDLs prevented the impairment of LTP caused by ADDLs (grey triangles, 151±9%,n=6,P>0.05).Pvalues were calculated using one-way ANOVA and the Tukey–Kramerpost hoctest. (b) As inaabove, but ICSM-18 (which recognizes an epitiope within residues 143–153 of PrP) was used in place of ICSM-35. Like ICSM-35, ICSM-18 (grey triangles, 157±9%,n=6) completely ameliorated the inhibitory activity of ADDLs (P<0.01).#Refers to perfusion of ICSM18/35; *refers to perfusion of ADDLs; arrow denotes TB stimulation. Inset calibration: 1 mV, 5 ms, stimulus artefact was removed for clarity.Pvalues were calculated using one-way ANOVA and the Tukey–Kramerpost hoctest. (c) Synaptic field potentials were recordedin vivofrom the CA1 area of anaesthetized male Wistar rats. In vehicle-injected rats (#first injection 10 μl i.c.v.; *second injection 5 μl 30 min later), high-frequency stimulation (HFS) triggered persistent and stable LTP (black squares, 136±7% at 3 h post tetanus,n=5). In contrast, injection of 5 μl Aβ-containing brain extract 15 min before HFS, in animals pre-injected with an IgG1 isotype control antibody (30 μg), significantly inhibited LTP (red circles, 106±4%,n=5,P<0.05). Importantly, injection of the anti-PrPCantibody, ICSM-18 30 min before injection of Aβ-containing TBS AD brain TBS extract (15 min before HFS) prevented the inhibition of LTP (grey triangles, 136±5%,n=5). Calibration: 2 mV, 10 ms.#Refers to injection of ICSM18; *refers to injection of TBS extract of human-derived Aβ; arrow denotes HFS. Insets show representative electrophysiological traces at the times indicated before (1,3,5) and after (2,4,6) conditioning stimulation. Data represent mean±standard deviation and is the average ofn= 6 from six individual mice. Figure 4: Inhibition of LTP by ADDLs or Aβ-containing AD brain extract is ameliorated by the anti-PrP C antibodies ICSM-35 and ICSM-18. ( a ) Conditioning stimulation in hippocampal slices from C57Bl/6J mice treated with vehicle solution induced a robust LTP (black squares, 152±7%, n =6), whereas pretreatment (30 min) with ADDLs significantly depressed LTP (red circles, 115±5%, n =8, p<0.01). In contrast, perfusion of slices with the anti-PrP antibody, ICSM-35 (which recognizes an epitope within the residues 93–102; 2 μg ml −1 ), 20 min before application of ADDLs prevented the impairment of LTP caused by ADDLs (grey triangles, 151±9%, n =6, P >0.05). P values were calculated using one-way ANOVA and the Tukey–Kramer post hoc test. ( b ) As in a above, but ICSM-18 (which recognizes an epitiope within residues 143–153 of PrP) was used in place of ICSM-35. Like ICSM-35, ICSM-18 (grey triangles, 157±9%, n =6) completely ameliorated the inhibitory activity of ADDLs ( P <0.01). # Refers to perfusion of ICSM18/35; *refers to perfusion of ADDLs; arrow denotes TB stimulation. Inset calibration: 1 mV, 5 ms, stimulus artefact was removed for clarity. P values were calculated using one-way ANOVA and the Tukey–Kramer post hoc test. ( c ) Synaptic field potentials were recorded in vivo from the CA1 area of anaesthetized male Wistar rats. In vehicle-injected rats ( # first injection 10 μl i.c.v. ; *second injection 5 μl 30 min later), high-frequency stimulation (HFS) triggered persistent and stable LTP (black squares, 136±7% at 3 h post tetanus, n =5). In contrast, injection of 5 μl Aβ-containing brain extract 15 min before HFS, in animals pre-injected with an IgG1 isotype control antibody (30 μg), significantly inhibited LTP (red circles, 106±4%, n =5, P <0.05). Importantly, injection of the anti-PrP C antibody, ICSM-18 30 min before injection of Aβ-containing TBS AD brain TBS extract (15 min before HFS) prevented the inhibition of LTP (grey triangles, 136±5%, n =5). Calibration: 2 mV, 10 ms. # Refers to injection of ICSM18; *refers to injection of TBS extract of human-derived Aβ; arrow denotes HFS. Insets show representative electrophysiological traces at the times indicated before (1,3,5) and after (2,4,6) conditioning stimulation. Data represent mean±standard deviation and is the average of n = 6 from six individual mice. Full size image Having found that anti-PrP antibodies prevented ADDL-mediated inhibition of LTP in mouse hippocampal slices, next we examined the in vivo efficacy of one of the antibodies, ICSM-18, in a different species, the rat. This would confirm if the PrP-dependence of Aβ toxicity was species, as well as mouse strain, independent. We directly compared the ability of ICSM-18 with an IgG1 isotype control antibody to abrogate the inhibition of hippocampal LTP by the pathophysiologically relevant Aβ-containing TBS extract of AD brain. In addition, to confirm that the involvement of PrP was not limited to extracts from a single AD brain, we used extracts from different AD and control brains than those used in Figure 2d . Intracerebroventricular (i.c.v.) pre-injection of the anti-PrP antibody completely prevented the AD brain Aβ-mediated inhibition of high-frequency stimulation (HFS)-induced LTP. In contrast, animals injected with AD brain extract immunodepleted of Aβ ( Supplementary Fig. S7 ) no longer blocked LTP (131±6, n =6; P <0.05 compared with baseline, paired t -test; P >0.05 compared with vehicle-injected controls at 3 h, one-way ANOVA, data not shown). Thus, acute administration of soluble extract from AD brain (5 μl, i.c.v. ; Fig. 4c ) completely inhibited LTP at 3 h post-HFS in an Aβ-dependent manner in animals injected 30 min previously with the control antibody (30 μg in 10 μl, i.c.v. ; P >0.05 compared with baseline, paired t -test; P <0.05 compared with controls that received two vehicle injections, one-way ANOVA). In contrast, in animals that were pre-injected i.c.v. with ICSM-18 (30 μg) HFS induced robust LTP ( P <0.05 compared with baseline (paired t -test) and compared with AD brain Aβ+control IgG1, one-way ANOVA) that was similar in magnitude to controls ( P >0.05, one-way ANOVA). When injected alone, neither ICSM 18 nor the control IgG1 significantly affected the magnitude of LTP ( Supplementary Fig. S6c ). The finding that sequence-selective targeting of PrP using antibodies can ameliorate the plasticity-impairing activity of AD brain-derived material in rats in vivo corroborates our in vitro finding with ADDLs and strongly encourages further exploration of this approach as an attractive therapeutic strategy. These data support the earlier finding that PrP C functions as a receptor for mediating toxicity of certain Aβ species. That the inhibitory effect of ADDLs on synaptic plasticity is PrP C -dependent has been confirmed using in vitro LTP recordings from congenic wild-type and PrP null mice and importantly that PrP expression is required for the plasticity-impairing activity of human brain-derived Aβ. There has been much debate about the nature of biologically relevant Aβ oligomers. Here we used two distinct preparations, one prepared from synthetic Aβ 1−42 to form ADDLs, and which we were careful to confirm to be biologically active and the other derived from the water-soluble phase of human AD brain. By using ADDLs, which are known to be active and to have similar biophysical characteristics as those used by Lauren et al, we could test the veracity of earlier reports that Aβ toxicity was mediated (at least in part) through PrP. Importantly, both preparations inhibited LTP in a PrP-dependent manner, suggesting that the ADDL preparation contained a component with similar properties to those found in AD brain. Heterogeneous preparations of Aβ aggregates are known to have nonspecific cytotoxicity at high concentrations and it would therefore be incorrect to interpret a failure of PrP targeting to ameliorate such nonspecific toxicity as excluding a role for PrP in Aβ-mediated neurotoxicity. Therefore, to expect PrP ablation to block toxicity in all aspects of all models would be to oversimplify a complex problem. The dependence of toxicity on particular receptors in individual animal models of AD may allow us to ascertain which models correctly mimic particular aspects of AD. A number of synaptic proteins have been shown to affect the binding and toxic effects of Aβ. mGluR5 was shown to affect binding of Aβ oligomers to excitatory synapses with anti-mGluR5 antibodies reducing Aβ oligomer binding by 50% (ref. 28 ). This is a similar level of reduction shown by PrP [6] . Although the affect of this receptor on Aβ binding was directly visualized, a binary interaction between Aβ and mGluR5 has not been proven. EphB2 was recently shown to co-precipitate with cell-derived Aβ and the fibronectin-repeat domain was shown to be critical [29] . Again, a direct binary interaction has not been proven. The LTP deficit in the J20 mouse model of AD, caused by downregulation of N -methyl- D -aspartate receptor, was reversed by overexpressing EphB2 and it would be interesting to see if this also applies to exogenous human brain-derived Aβ or whether this requires in situ Aβ present over longer periods. Previous studies have shown N -methyl- D -aspartate receptor are involved in toxic effects related to ADDLs but appear not to bind directly [30] . Given that PrP has been suggested to interact with NR2D subunits and attenuate excitotoxicity [31] it is plausible that a number of these proteins are involved in Aβ toxicity through similar pathways. In that sense, the lack of a vital PrP function would make it a most attractive therapeutic target. In addition, the demonstration that Aβ-mediated inhibition of LTP in vivo and in vitro can be blocked by anti-PrP antibodies further extends these findings, arguing against the effect in PrP null mice being due to unknown protective effects of constitutive PrP ablation. That antibodies raised against two structurally and sequentially different regions of the protein are active strongly argues that PrP is the target of these antibodies in vivo and that the effect is not nonspecific. Furthermore, these same antibodies have already been used to successfully treat prion disease in mice without causing toxic effects [15] . The PrP:Aβ-binding interaction has been further characterized using material of known biological activity and a biophysical assay developed to investigate potential therapeutic agents, which might efficiently disrupt this interaction. The anti-PrP monoclonal antibodies ICSM-18 and 35, already extensively studied in vivo in mouse and fully humanized for investigation as putative human anti-prion therapeutics, potently inhibit Aβ-induced effects on synaptic plasticity both in vitro and in vivo suggesting that the humanized versions of these antibodies should be considered for potential AD therapeutic trials either individually or in combination. As both ADDL preparations and Aβ extracted from human brain in aqueous buffer are highly heterogeneous, additional studies are required to biophysically characterize the key toxic species that bind to PrP. Materials Aβ 1−42 was from California Peptide Research and biotinylated Aβ 1−42 with biotin attached to Asp1 using a 6-carbon linker (bAβ 1−42 ) was synthesized, and purified by Dr James I. Elliott at Yale University (New Haven, CT). Peptide masses and purities were determined by electrospray ionization/ion trap mass spectrometry and reverse-phase HPLC, respectively. Other reagents were purchased from Sigma Aldrich unless otherwise stated. Production of ADDL and bADDL preparations bAβ 1−42 or Aβ 1−42 ( ∼ 1.25 mg) was dissolved in HFIP, sonicated and left to stand at room temperature for 1 h. The HFIP was evaporated under a stream of dry air/N 2 to produce a clear film. The peptide film was dissolved in anhydrous dimethylsulphoxide (DMSO) with vigorous vortexing then diluted to 100 μM in phenol red-free Ham's F12 medium (Promocell GmbH) and vortexed for 15 s. Samples were incubated at room temperature for 16 h. Finally, samples were centrifuged at 14,200 g for 15 min, used immediately or snap frozen in liquid N 2 and stored at −80 °C. Monomeric Aβ 1−42 was produced by dissolving Aβ 1−42 peptide in 10 mM NaOH (pH 11) for 1 h. Size-exclusion chromatography Aliquots (0.5 ml) of freshly prepared 100 μM Aβ 1−42 (10 mM NaOH, pH 11), ADDLs and bADDLs (phenol red-free Ham's F12 medium, 2% DMSO) were injected onto a Superdex 75 10/30 column (GE Healthcare) and eluted with PBS at a flow rate of 0.8 ml min −1 using an AKTA FPLC and peptide eultion monitored by absorbance at 280 nm. Sedimentation velocity analytical ultracentrifugation Experiments were performed on a Beckman XLI analytical ultracentrifuge (Beckman). Freshly prepared 100 μM bADDLs (phenol red-free Ham's F12 medium, 2% DMSO) were centrifuged at 201,600 g at 20 °C with absorbance data collected at 278 nm. Sedimentation velocity data were analysed as described [32] , [33] and graphically presented in the standard format with the sedimentation coefficient plotted against the sedimentation coefficient distribution. Electron microscopy For analysis, a 4 μl drop of bADDLs/ADDLs was loaded onto negatively glow discharged copper grids, which had been previously coated with a continuous carbon film. The sample was left to adhere for 30 s and excess solution carefully blotted using grade 4 Whatman paper, the sample stained with 2% uranyl acetate (6 μl) for 30 s, blotted and the grid left to air dry. Images were recorded on film at a magnification of ×42,986 using an FEI Tecnai T12 EM operating at 120 kV. Imaging was done at a defocus range of 700 nm to 1 μm and an electron dose of 10–20 electrons per Å 2 . Films were digitized with a step size of 7 μm using a Zeiss SCAI film scanner, giving a pixel size of 1.63 Å. SDS–PAGE Aliquots (5 & 10 μl) of 10 μM bADDL and ADDL preparations were boiled in sample buffer and electrophoresed on 16% polyacrylamide Tris–tricine gels and analysed for Aβ content by comparison to known Aβ standards following visualization by silver staining. Alternatively, the ADDLs/bADDLS were diluted to 1:10 (1 μM) in sample buffer and used without boiling for western blotting with the amino-terminal anti-Aβ antibody, 6E10 (Signet). Immunoreactive bands were detected and quantified using a Licor Odyssey imaging system (Licor Biosciences). Preparation of human AD brain samples All procedures for use of human tissue in this research were approved by a multicentre Research Ethics committee. Three brain samples were used for this study: one from a 78-year-old female with a history of dementia and confirmed Alzheimer's disease pathology (from Asterand), a second from an 80-year-old female (Queen Square Brain Bank for Neurological Disorders, UCL Institute of Neurology) with clinical and pathological diagnoses of AD and the other from a cognitively intact 68-year-old female (Queen Square Brain Bank for Neurological Disorders, UCL Institute of Neurology). Samples of frozen posterior temporal cortex were used to prepare water-soluble Aβ homogenates free from membrane-bound or plaque-associated material. The homogenates were dialysed at 4 °C and stored at −80 °C .The amount and form of Aβ present was determined by western blotting and quantified by comparison to synthetic Aβ standards [34] . Generation of FVB/N congenic PrP knockout line The FVB/N- Prnp o/o (PrP null) congenic line was generated by ten generations of backcrossing ZH1 PrP null mice [35] to FVB/N followed by genetic testing by Charles River (Margate, UK) using 84 FVB-specific PCR microsatellite makers covering 19 chromosomes at ∼ 20 cM intervals to select breeding pairs positive for 100% of the FVB-specific markers. The selected congenic pairs were inter-bred to remove the endogenous murine PrP gene and to restore homozygosity of the knockout allele. In vitro electrophysiology Two- to four-month-old FVB/N (Harlan, Wyton, UK) or PrP null mice (FVB/N- Prnp o/o , MRC Prion Unit) were used to study the effects of bADDLs and Aβ-containing extracts of human brain. In addition, 2- to 3-month-old C57BL/6J mice (Charles River, Margate, UK) were used to examine the effects of bADDLs/ADDLs and the anti-PrP antibodies, ICSM-18 and ICSM-35. Male mice were used in all experiments to eliminate any gender bias and were group housed under normal 12-h light–dark conditions. In all cases, mice were anaesthetized with isoflurane/O 2 and decapitated. The brain was rapidly removed and immersed in ice-cold sucrose-based artificial cerebrospinal fluid before parasagital sections (350 μm) were prepared on a Leica VT1000S vibratome (Leica). Slices were allowed to recover for at least 90 min before being submerged in a recording chamber and perfused with oxygenated artificial cerebrospinal fluid at 30 °C. Extracellular field excitatory postsynaptic potentials (fEPSPs) were recorded from stratum radiatum of area CA1 of the hippocampus. Following baseline recording, LTP was induced by theta-burst stimulation (ten bursts of four stimuli at 100 Hz, with an interburst interval of 200 ms) given at baseline intensity. In experiments using bADDLs/ADDLs or TBS extracts of human brain, the sample was added to the perfusate 30 min before induction of LTP. Where a combination of ADDLs and anti-PrP antibodies were used, the antibody was added to the perfusate 20 min before the ADDLS. Once added to the perfusate, ADDLs, brain samples and/or antibodies were present for the duration of the experiment. In vivo electrophysiology In vivo studies on urethane (1.5 gm kg −1 intraperitoneal) anaesthetized male adult Wistar rats (250–300 g) were approved by Trinity College Dublin's Ethical Review Committee and by the Department of Health, Republic of Ireland. Single-pathway recordings of fEPSPs were made from the stratum radiatum in the CA1 area of the right hippocampal hemisphere in response to stimulation of the ipsilateral Schaffer collateral-commissural pathway. Test fEPSPs were evoked at a frequency of 0.033 Hz and at a stimulation intensity adjusted to elicit a fEPSP amplitude of 50% of maximum. LTP was induced following a HFS consisting of 10 bursts of 20 stimuli with an inter-stimulus interval of 5 ms (200 Hz), and an inter-burst interval of 2 s. A stainless-steel guide cannula was implanted above the right lateral ventricle to allow i.c.v. injection of human brain samples, control solution and/or anti-PrP antibody (ICSM18). Verification of the placement of the cannula was performed post-mortem by checking the spread of i.c.v.-injected ink dye. Protein expression and purification Constructs of human PrP were expressed [36] and purified [37] as described previously. Protein quality was confirmed by SDS–PAGE, MALDI–TOF mass spectrometry and circular dichroism spectroscopy. DELFIA Human PrP (10 mM sodium carbonate, pH 9.6) was bound to medium binding 96-well white plates (Greiner) and blocked with BSA. If required, antibody was then incubated for 1 h. Different preparations of Aβ 1−42 were incubated for 1 h. Aβ was detected by 6E10 for 1 h and incubated for 30 min with DELFIA Eu-N1 anti-mouse antibody before enhancing with DELFIA enhancement solution [38] . Biotinylated Aβ was detected by DELFIA Eu-N1 streptavidin before enhancing with DELFIA enhancement solution. For PrP antibody-binding experiments, ICSM antibodies (D-Gen Ltd) were incubated for 30 min with DELFIA Eu-N1 anti-mouse antibody before enhancing with DELFIA enhancement solution. Binding of antibodies to PrP was detected by incubation for 30 min with DELFIA Eu-N1 anti-mouse antibody before enhancing with DELFIA enhancement solution. Plates were scanned for time-resolved fluorescence intensity using a Perkin-Elmer EnVision plate reader (Perkin-Elmer). Binding constants were calculated using a 1-site Langmuir isotherm and were tested for tight-binding characteristics. This ensures a true K d can be measured and that direct saturation of the protein surface as soon as stoichiometric quantities of peptide are added has not occurred. Molecular modelling A model of the full ISCM-18 antibody complex with human PrP C 119−231 was constructed by superimposing PrP-Fab complex (2W9E) onto the Fab domains of a full human IgG antibody structure (1HZH). The ADDL particle was constructed as described in the Supplementary Methods . The N-terminus of the PrP C molecule, taken from the Fab crystal structure complex (2W9E), was extended back to residue 95 as an unstructured polypeptide. Copies of this molecule were manually docked to the surface of the ADDL particle. Molecular graphics and model building were performed using InsightII (2005) and energy calculations using Discover 2.98 (Accelrys). Full methods describing the preparation of ADDL/bADDL, human AD brain samples, the in vitro and in vivo electrophysiology, DELFIA and molecular modelling can be found in the Supplementary Methods . How to cite this article: Freir, D.B. et al . Interaction between prion protein and toxic amyloid β assemblies can be therapeutically targeted at multiple sites. Nat. Commun. 2:336 doi: 10.1038/ncomms1341 (2011).